Fractional Bloch oscillations in photonic lattices Bloch oscillations, the oscillatory motion of a quantum particle in a periodic potential, are one of the most fascinating effects of coherent quantum transport. Originally studied in the context of electrons in crystals, Bloch oscillations manifest the wave nature of matter and are found in a wide variety of different physical systems. Here we report on the first experimental observation of fractional Bloch oscillations, using a photonic lattice as a model system of a two-particle extended Bose–Hubbard Hamiltonian. In our photonic simulator, the dynamics of two correlated particles hopping on a one-dimensional lattice is mapped into the motion of a single particle in a two-dimensional lattice with engineered defects and mimicked by light transport in a square waveguide lattice with a bent axis. Bloch oscillations (BO), that is, the oscillatory motion of a quantum particle in a periodic potential driven by a constant force, constitute one of the most striking and oldest predictions of coherent quantum transport in periodic lattices [1] , [2] . In natural crystals, BO have never been observed because of dephasing effects. Solely with the advent of semiconductor superlattices and ultracold atoms, BO have been observed for matter waves [3] , [4] , [5] , [6] . In their essence, BO are a wave phenomenon. As such, they are found for optical [7] , [8] , [9] , [10] , [11] and acoustic [12] waves as well. When interactions between particles compete with their mobility, novel dynamical behaviour can arise where particles form bound states [13] and co-tunnel through the lattice [14] . While particle interaction has been generally associated to BO damping [15] , [16] , [17] , for few strongly interacting particles it was predicted that bound states undergo fractional BO at a frequency twice (or multiple) that of single-particle BO [18] , [19] , [20] . The observation of fractional BO is challenging in condensed-matter systems and up to now has not been achieved even in model systems. Ultracold quantum gases in optical lattices have provided in the past decade a powerful laboratory tool to simulate Hubbard models of condensed-matter physics [21] . Experiments with ultracold atoms have so far demonstrated the existence of bound-particle states and correlated tunnelling phenomena [13] , [14] , however fractional BO of atomic pairs have not been observed yet. A photonic simulator of the Hubbard model can map the dynamics of two correlated particles hopping on a one-dimensional (1D) lattice into the motion of a single particle in a 2D lattice with engineered defects [22] , [23] , thereby offering the possibility to easily visualize the effect under simulation, but requiring a high level of control of the photonic structure. Here we report on the first observation of fractional BO using a photonic lattice as a model system of a few-particle extended Bose–Hubbard Hamiltonian, which is the most appropriate theoretical framework to consistently describe fractional BO. Theory of BO in the extended Bose–Hubbard (EBH) model To study correlated BO, we consider an EBH model [24] , [25] , [26] describing strongly interacting bosons in the lowest Bloch band of a 1D lattice driven by an external force. This model is more accurate than the standard BH model as it accounts for higher-order processes whose magnitude is comparable with the one of second-order tunnelling [26] . The Hamiltonian of the system is given by Ĥ = Ĥ EBH + Ĥ F , where describes the effect of the external constant force F ( d is the lattice period) and is the EBH Hamiltonian. Ĥ EBH includes the standard BH Hamiltonian (with ħ =1) and three additional terms [24] , whose explicit expression is given in Supplementary Note 1 . In equation (1), U 0 is the on-site energy interaction strength ( U 0 >0 for a repulsive interaction); J is related to the single-particle hopping rate between adjacent lattice sites; is the lattice attenuation factor [24] ; and are the bosonic creation and annihilation operators and is the particle number operator at lattice site l . The standard BH term Ĥ BH describes on-site particle–particle interaction and single-particle tunnelling between adjacent lattice sites ( Fig. 1a ). The additional terms Ĥ 3 , Ĥ 4 and Ĥ 5 account for nearest-neighbor hopping of single atoms conditioned by the on-site occupation number, nearest-neighbor interactions, and nearest-neighbor hopping of bosonic pairs, respectively ( Fig. 1c ). 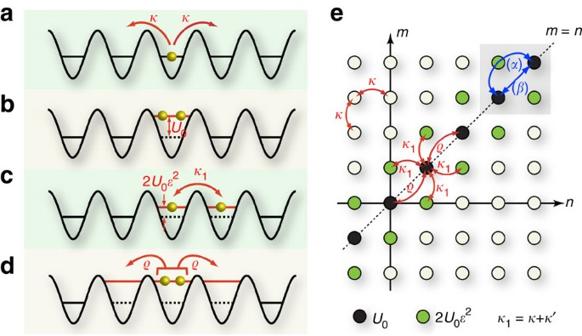Figure 1:Dynamics of two interacting bosons in the extended Bose–Hubbard lattice. Two-particle dynamics in the EBH model: (a) Single-particle tunnelling; (b) on-site particle interaction; (c) nearest-neighbor-site particle interaction and conditional single-particle tunnelling; (d) nearest-neighbor hopping of particle pairs. (e) Fock-space representation of the two-particle dynamics; the upper-right inset represents the two possible pathways for two-particle hopping to the nearest-neighbor site: (α) is the second-order pair tunnelling, while (β) is the direct two-particle tunnelling. Figure 1: Dynamics of two interacting bosons in the extended Bose–Hubbard lattice . Two-particle dynamics in the EBH model: ( a ) Single-particle tunnelling; ( b ) on-site particle interaction; ( c ) nearest-neighbor-site particle interaction and conditional single-particle tunnelling; ( d ) nearest-neighbor hopping of particle pairs. ( e ) Fock-space representation of the two-particle dynamics; the upper-right inset represents the two possible pathways for two-particle hopping to the nearest-neighbor site: ( α ) is the second-order pair tunnelling, while ( β ) is the direct two-particle tunnelling. Full size image In the absence of particle interaction, each particle undergoes independent BO on the lattice. The single-particle amplitude probabilities A n ( t ) to find the particle at lattice site n evolve according to the coupled equations where κ = ɛJ /2 is the single-particle hopping rate. The single-particle energy spectrum is given by an equally spaced Wannier–Stark ladder [27] , [28] , which is the spectral counterpart of BO and results in a periodic dynamics at the frequency ω B = Fd . For single-site excitation, that is, , BO appear as a breathing (rather than an oscillatory) motion at the frequency ω B . Photonic demonstrations of such BO breathing dynamics were previously reported in refs 7 , 8 , 10 . Let us now consider the dynamics of two interacting particles. The state vector of the system can be expanded in Fock space as , where c n,m ( t ) is the amplitude probability to find one particle at site n and the other particle at site m , with c n,m = c m,n for bosons. The evolution equations for the amplitude probabilities ( Supplementary Note 2 ) show that the dynamics of the two correlated bosons on the 1D lattice can be mapped into the motion of a single-particle hopping on the 2D square lattice of Fig. 1e . The square lattice shows both energy site defects and hopping rate corrections on the three diagonals m = n , n ±1. Far from the main diagonal, the square lattice is homogeneous with a uniform hopping rate κ = ɛJ /2, which is the single-particle hopping rate of the original problem ( Fig. 1a ). The site energy defects U 0 and on the main ( m = n ) and nearest-neighbor ( m = n ±1) diagonals account for on-site and nearest-neighbor-site particle repulsion, respectively ( Fig. 1b ). The correction of hopping rates (with ) on the main diagonal accounts for nearest-neighbor hopping of single atoms conditioned by the on-site occupation number ( Fig. 1c ). Finally, the cross coupling on the main diagonal n = m describes nearest-neighbor hopping of bosonic pairs, that is, direct two-particle tunnelling ( Fig. 1d ). These additional terms could degrade BO and therefore their effect has been carefully investigated ( Supplementary Note 2 ). It can be shown that for two strongly correlated particles ( ), only the direct two-particle tunnelling is important, competing with second-order pair tunnelling. In fact, let us assume as an initial condition , that is, the two particles are initially placed on the same site, with a probability to find both particles at site n . Then an asymptotic analysis of the underlying equations shows that the two particles form a bound state, that is they co-tunnel along the lattice, undergoing BO at the frequency 2 ω B =2 Fd twice the single-particle BO frequency ω B . In Fock space, this means that we expect to observe, along the main diagonal m = n of the square lattice of Fig. 1e , periodic revivals at frequency 2 ω B . Precisely, as shown in the Supplementary Note 2 (see also the Supplementary Figs S1 and S2 ), the bound-particle occupation amplitudes at the various lattice sites evolve according to equation (2), but with F replaced by 2 F and κ replaced by κ eff . The effective hopping rate of the bound-particle state, , includes second-order tunnelling (−2 κ 2 / U 0 ) and direct two-boson tunnelling ( ρ ) processes. Such two contributions always add with the same sign, for both repulsive ( U 0 >0) and attractive ( U 0 <0) interactions, and generally are of the same order of magnitude. The bound-particle state thus behaves like a single particle hopping on the 1D lattice, but with a driving force which is doubled as compared with that of a single particle [18] , [19] and with a modified hopping rate κ eff . Note that the effect of direct two-atom tunnelling on the BO dynamics, not considered in previous works [19] , [20] , [22] , is to increase the amplitude of the breathing motion (owing to the correction of κ eff ), whereas the periodicity of the BO is preserved. Experimental photonic simulator In our experiments, single-particle hopping dynamics in the square lattice of Fig. 1e has been simulated by discretized spatial light transport in an engineered 2D square lattice of evanescently coupled optical waveguides [29] . This lattice has been fabricated in a fused silica substrate by direct waveguide writing with femtosecond lasers [30] , [31] , [32] , [33] , [34] , taking advantage of the 3D capabilities of this technology. The spatial propagation of the light intensity in the generic ( m,n )-th lattice site maps the temporal evolution of the two-particle probability distribution in Fock space [29] , [33] . In the photonic simulator of Ĥ EBH , the role of the hopping coefficients κ and ρ is played by the evanescent coupling constants between first- and second-neighbouring waveguides ( and ), respectively. The former is in general greater than the latter and the relative weight can be tuned by properly engineering the lattice parameter d ( Supplementary Note 3 and Supplementary Fig. S3b,c ). The on-site particle-interaction defect U 0 is realized by fabricating the main diagonal waveguides with a different refractive index change (this is achieved by slightly modifying the writing speed of the waveguides, as discussed in the Supplementary Note 3 and illustrated in the Supplementary Fig. S3a ) and thus with the propagation constant β ′ slightly detuned with respect to that of all the others ( β ). The positive or negative sign of the relative detuning Δ β=β − β ′ determines the repulsive or attractive nature of the interaction, respectively. Lastly, we did not add any special feature in the nearest-neighbouring diagonals, because, as already discussed above, the nearest-site effects described in Fig. 1c are negligible with respect to the other terms of the EBH model. The implementation of the driving force term Ĥ F is obtained by a constant bending of the waveguide axes (radius of curvature R , ) in the plane determined by the lattice main diagonal direction Y and the light propagation direction z ( [10] ). In Fig. 2a , the whole lattice structure is depicted. Note that the array cross-section is rotated in such a way that the bending plane is horizontal in the laboratory reference frame (45° rotation with respect to Fig. 1e) . This simplifies the fabrication process and the imaging of the light propagating in the waveguides; in this way, although being a 3D structure, each waveguide remains on a specific horizontal plane. 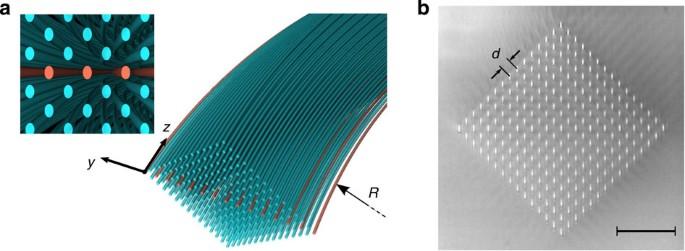Figure 2: The photonic simulator of correlated BO. (a) Sketch of the waveguide array structure; red-coloured waveguides have a different refractive index change with respect to the others to implement the on-site particle-interaction defectU0. (b) Section of the fabricated array, imaged with an optical microscope. Scale bar, 100 μm. Figure 2: The photonic simulator of correlated BO. ( a ) Sketch of the waveguide array structure; red-coloured waveguides have a different refractive index change with respect to the others to implement the on-site particle-interaction defect U 0 . ( b ) Section of the fabricated array, imaged with an optical microscope. Scale bar, 100 μm. Full size image In a first experiment, we checked that our photonic simulator can reliably mimic the dynamics governed by Ĥ EBH alone, namely without the action of the external constant force. For this purpose, we fabricated 225 straight waveguides ( ) arranged in a 15 × 15 square lattice, with spacing d =19 μm and a length L =2.5 cm. For such a lattice spacing, the coupling coefficients are and . To simulate particle interaction, we fabricated the main diagonal waveguides with a propagation constant detuning Δ β =−4 cm −1 , therefore representing an attractive interaction between the particles. A microscopic image of the array section is reported in Fig. 2b . We coupled 633 nm He-Ne laser radiation into the central waveguide, belonging to the main diagonal subset and thus corresponding to an initial condition where the two particles occupy the same lattice site. As previously discussed, light is expected to preferably remain on the detuned diagonal, representing the fact that the correlated particles will hop together to the next site and will hardly separate. To study the evolution of the system, we monitored the light propagation along the array by imaging from above the fluorescence light at 650 nm emitted from the waveguides and arising from colour centres created in the femtosecond laser-writing process. As the colour centres are formed exclusively inside the waveguides, this technique yields a high signal-to-noise ratio and permits a direct imaging of the light propagation in the waveguide arrays [33] , [34] . The result obtained in this first experiment is visible in Fig. 3a . The measured distribution of light in the photonic model implementing both contributions to the bound state hopping rate, that is, two-particle direct tunnelling and second-order pair tunnelling, is compared with the corresponding numerical simulation ( Fig. 3b ). The excellent agreement demonstrates that our photonic model can indeed take into account both contributions and thus correctly implements the EBH model. The role of the direct two-particle tunnelling ( Fig. 1d ), neglected in the standard BH model, can be quite relevant as shown by the different light distributions obtained from numerical simulations of the same structure but including only the second-order tunnelling ( Fig. 3c ). 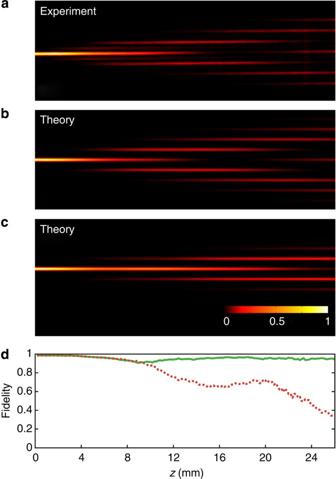Figure 3: Photonic simulation of the delocalization dynamics of two interacting particles in a lattice. (a) Experimental simulation in a waveguide lattice implementing direct two-particle tunnelling and second-order pair tunnelling with a similar weight. (b) Numerical simulation including both contributions (EBH model). (c) Numerical simulation including only second-order pair tunnelling (BH model). (d) Fidelity (see main text for definition) of the experimental light distribution with that predicted by the EBH model (continuous line) and with that predicted by the standard BH model (dotted line). Figure 3: Photonic simulation of the delocalization dynamics of two interacting particles in a lattice. ( a ) Experimental simulation in a waveguide lattice implementing direct two-particle tunnelling and second-order pair tunnelling with a similar weight. ( b ) Numerical simulation including both contributions (EBH model). ( c ) Numerical simulation including only second-order pair tunnelling (BH model). ( d ) Fidelity (see main text for definition) of the experimental light distribution with that predicted by the EBH model (continuous line) and with that predicted by the standard BH model (dotted line). Full size image To introduce a more quantitative comparison between the experimental light distribution in the array with the expected one, we introduce a metric, called fidelity, which provides the overlap between the experimental, I exp , and theoretical, , intensity profiles at each position z . Such metric is analytically defined as where Δ Y z indicates, at a given propagation distance z , the transverse coordinate interval Δ Y along which the intensity profile is considered. This metric ranges between 0 for completely uncorrelated profiles to 1 for perfect overlapping. We have calculated this function for the graphs in Fig. 3a–c and reported the results in Fig. 3d . Also from the quantitative point of view, it can be concluded that our photonic simulator is capable of faithfully implementing the EBH model, with an average fidelity as high as 95%. In addition, it can be observed how modelling the same phenomenon with a standard BH model provides quite different predictions already after a limited propagation length with a fidelity to the experimental results as low as 35% at the end of the device. A careful observation of Fig. 3a would reveal the presence of illuminated waveguides at interstitial positions with respect to the waveguide array at the detuned diagonal plane. These waveguides are actually at a different depth and belong to the first neighbouring plane. Their faint illumination (partially due to an out-of-focus condition) is nevertheless a clear indication that, due to the second-order pair tunnelling mechanism, light spreads also outside the main diagonal plane. Observation of fractional BO In a second experiment, we proceeded to the observation of fractional BO. To this purpose, we fabricated another 15 × 15 square waveguide lattice, with the same lattice spacing and detuning on the diagonal as in the previous structure. To mimic the external force F , the waveguides are now circularly bent with a radius R =400 cm, as depicted in Fig. 2a . The array length is L =8.5 cm. As in the previous experiment, we injected the probe light into the central waveguide and we imaged its propagation along the waveguide lattice diagonal (Y), where light is confined. 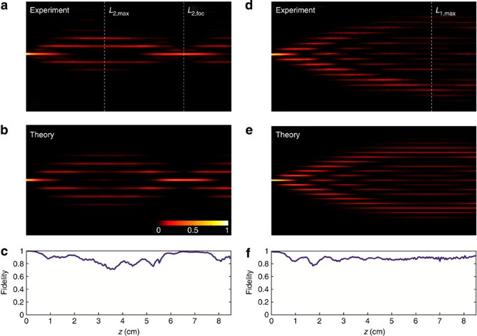Figure 4: Photonic simulation of BO for correlated and single particles. (a) Experimental and (b) numerical images of the light intensity distribution in the waveguide lattice main diagonal versus propagation distancez, representing in Fock space the BO for two interacting particles. Inc, the evolution of the fidelity, as given by equation (3), is also shown. (d–f): same as (a–c), but for the single-particle BO in the 1D waveguide array. Note that in this case, the position where the BO amplitude is at maximum (L1,max) corresponds to the refocusing condition for the two-particle BO (L2,foc=L1,max=6.5 cm). Figure 4a shows the oscillatory behaviour of the light dynamics along the waveguide array. Initially, light spreads into several waveguides, until it reaches a maximum of the breathing amplitude (around L 2,max =3.25 cm). Then light refocuses into the central waveguide ( L 2,foc =6.5 cm) and the breathing starts again. This periodic behaviour represents the correlated BO of two interacting particles, watched in Fock space. The accuracy of the fabricated photonic simulator is confirmed by the very good agreement with the numerical simulations of light propagation in the designed structure ( Fig. 4b ). A quantitative estimation of the agreement is provided by the fidelity, reported in Fig. 4c , that yields an average value of 90%. To better analyse this result, we cut the sample at L 2,max and L 2,foc and we imaged onto a CCD camera the light distribution exiting the output facet of the array ( Fig. 5 ). 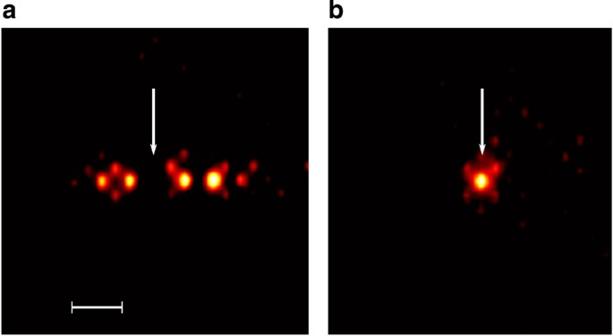Figure 5: Output light distribution at two propagation lengths. Measured light distribution in the waveguide lattice section (corresponding toFig. 4a) at positions (a)L2,max, where the fractional BO amplitude is at maximum and (b)L2,focwhere light refocuses to the initial waveguide (indicated by a white arrow in both panels). Scale bar, 50 μm. Figure 5a clearly shows that, even in correspondence of the breath maximum amplitude, light remains mainly confined in the waveguide lattice-detuned diagonal. This fact is a further demonstration that two interacting particles, initially in the same lattice site, form a bound state and hop together to neighbouring sites. Figure 5b shows that at the refocusing distance, all the light is indeed confined in the central waveguide, which was the one originally excited (indicated by a white arrow in both panels). A numerical simulation of the end-view distribution of light in the 2D array along the whole propagation length ( Supplementary Movie 1 ) confirms the experimentally observed pattern. Figure 4: Photonic simulation of BO for correlated and single particles. ( a ) Experimental and ( b ) numerical images of the light intensity distribution in the waveguide lattice main diagonal versus propagation distance z , representing in Fock space the BO for two interacting particles. In c , the evolution of the fidelity, as given by equation (3), is also shown. ( d – f ): same as ( a – c ), but for the single-particle BO in the 1D waveguide array. Note that in this case, the position where the BO amplitude is at maximum ( L 1,max ) corresponds to the refocusing condition for the two-particle BO ( L 2,foc = L 1,max =6.5 cm). Full size image Figure 5: Output light distribution at two propagation lengths. Measured light distribution in the waveguide lattice section (corresponding to Fig. 4a ) at positions ( a ) L 2,max , where the fractional BO amplitude is at maximum and ( b ) L 2,foc where light refocuses to the initial waveguide (indicated by a white arrow in both panels). Scale bar, 50 μm. Full size image The ‘fractional’ nature of BO for correlated particles can be appreciated by comparing Fig. 4a with the BO pattern for single-particle hopping in the same lattice under the action of the same force F , shown in Fig. 4d . We fabricated a planar 1D array of 23 identical waveguides, equally spaced of d ′= d =19 μm, and uniformly bent in the array plane with a constant radius of curvature R ′. Such a structure reliably simulates the dynamics of single particle BO [10] . To implement the same force on the single particle, we have to project the curvature on the diagonal for the two-particles structure on one of the main axis of the square lattice: this yields a curvature radius for the linear array . We imaged the light propagation in this waveguide array for a length L =8.5 cm ( Fig. 4d ). Also in this case, we observe a breathing propagation pattern corresponding to the single-particle BO, but the position of the maximum breath amplitude L 1,max corresponds to the refocusing position L 2,foc for two-particles BO ( Fig. 4a ). This demonstrates that the frequency of a two-particles BO is twice that for a single-particle. It may be worth noting that the breathing amplitude of a single-particle BO is larger than that for the two-particle BO. This is due to a higher hopping rate in the former case, κ > κ eff , and to the double force experienced by the two strongly correlated particles with respect to the single one. The agreement between the experimental light distribution ( Fig. 4d ) and the theoretical one ( Fig. 4e ) is reported in Fig. 4f in terms of fidelity, yielding an average value of 90%. We have experimentally observed the photonic quantum analogy of fractional BO of two strongly correlated particles. The Fock space dynamics of the two-particle EBH Hamiltonian is mapped into spatial propagation of discretized light in an engineered square lattice of evanescently coupled optical waveguides. We have experimentally verified the doubling of the BO frequency of correlated particles with respect to that observed for a single particle, and shown the competition of second-order tunnelling and direct two-particle tunnelling. The simple visualization of the phenomenon and the high control of the fabricated structure make our photonic model system a very powerful tool to investigate exotic non-equilibrium phenomena associated to the formation of particle-bound states that are difficult to access or prepare in the matter. It is envisaged that our model system could offer the possibility to visualize other intriguing phenomena involving few correlated particles, such as the interplay between particle interaction and Anderson localization [35] , [36] , quantum billiards and transition to quantum chaos [23] , anyonic BO [37] , correlated barrier tunnelling and particle dissociation [38] . Fabrication of the waveguide arrays Waveguide arrays have been fabricated by femtosecond laser waveguide writing in fused silica samples. The second harmonic of a HighQLaser femtoREGEN Yb-based amplified laser system has been used, consisting in 400-fs pulses at 520-nm wavelength with repetition rates up to 960 kHz. Actual writing conditions consisted of 300-nJ pulses delivered at a repetition rate of 20 kHz. Optimal range for the writing speed was identified as 8–14 mm s −1 , yielding propagation losses of about 0.5 dB cm −1 . To implement the detuning in the lattice diagonal, we modulated the writing speed, therefore the waveguides on the diagonal were fabricated at a speed of 9 mm s −1 , while all the others were written at 14 mm s −1 . The variation in writing speed modifies the propagation constants of the guided modes, producing the designed detuning Δ β =−4 cm −1 , but has a negligible effect on the coupling rate between the waveguides. End faces of the substrates were polished after laser writing to improve light launching and output imaging. Characterization of the light distribution in the arrays Femtosecond laser writing in fused silica creates colour centres that provide fluorescent emission at about 650 nm, when light at 633 nm is propagated in the waveguide. Top-view imaging of the fluorescence signal is employed to visualize and quantitatively estimate the light distribution along the waveguide array, rejecting the background light by a notch filter at 633 nm. Light collection for the top-view images is performed with a × 10 objective, 0.25 numerical aperture, placing the detuned diagonal at focus. The waveguides in the neighbouring planes go progressively out of focus, as the distance between planes is 13.5 μm and the Rayleigh range of the collecting optics is z R =4.6 μm; however, the first neighbouring plane of waveguides is still faintly visible in some of the images. To achieve a high resolution in imaging the light in the waveguide array all along its length, several images have been acquired and then stitched together. Propagation losses in the waveguides have been compensated by renormalizing the intensity levels in the acquired images. How to cite this article: Corrielli, G. et al . Fractional Bloch oscillations in photonic lattices. Nat. Commun. 4:1555 doi: 10.1038/ncomms2578 (2013).